Pd(II)-catalysedmeta-C–H functionalizations of benzoic acid derivatives Benzoic acids are highly important structural motifs in drug molecules and natural products. Selective C–H bond functionalization of benzoic acids will provide synthetically useful tools for step-economical organic synthesis. Although direct ortho -C–H functionalizations of benzoic acids or their derivatives have been intensely studied, the ability to activate meta -C–H bond of benzoic acids or their derivatives in a general manner via transition-metal catalysis has been largely unsuccessful. Although chelation-assisted meta -C–H functionalization of electron-rich arenes was reported, chelation-assisted meta -C–H activation of electron-poor arenes such as benzoic acid derivatives remains a formidable challenge. Herein, we report a general protocol for meta -C–H olefination of benzoic acid derivatives using a nitrile-based sulfonamide template. A broad range of benzoic acid derivatives are meta -selectively olefinated using molecular oxygen as the terminal oxidant. The meta -C–H acetoxylation, product of which is further transformed at the meta -position, is also reported. Benzoic acids are highly valuable structural motifs and precursors for synthesizing other organic substances. Direct and selective transformation of the C–H bonds of this class of compounds would be very attractive for developing step-economical organic syntheses ( Fig. 1 ) [1] , [2] , [3] , [4] , [5] , [6] , [7] , [8] , [9] , [10] , [11] , [12] , [13] , [14] . To date, direct ortho -C–H functionalizations of benzoic acids or their derivatives have been intensely studied with transition-metal catalysts [1] , [2] , [3] , [4] , [5] , [6] , [7] , [8] , [9] , [10] , [11] , [12] or by directed ortho metalation [13] . Traditionally, the meta -position of benzoic acids were functionalized by electrophilic aromatic substitution, which often requires harsh conditions as benzoic acids are generally deactivated towards this reaction [14] . Transition-metal catalysts have been used to functionalize meta -C–H bonds of limited benzoic acid derivatives. Hartwig, Yu, Sanford and others have achieved modest to high selectivity because of substrate steric or electronic control [15] , [16] , [17] , [18] , [19] , [20] , [21] , [22] , [23] , [24] , [25] . In prior examples, an excess of the benzoic acid derivative, which was often used as the solvent, was generally required with a Pd catalyst ( Fig. 1a ) [17] , [18] , [21] . Despite these highly important pioneering studies, the ability to activate the meta -C–H bond of benzoic acids or their derivatives in a general manner via transition-metal catalysis has been largely unsuccessful [25] . Therefore, a general approach to meta -C–H functionalization of benzoic acids or their derivatives regardless of the substitution patterns is highly desirable to provide synthetic short-cuts. 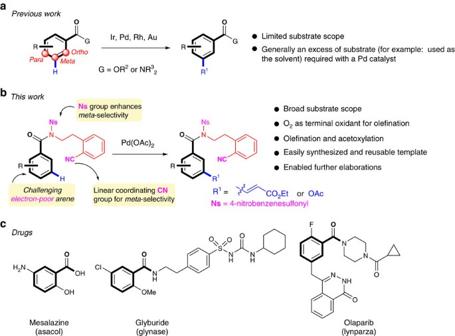Figure 1: Transition-metal-catalysedmeta-C–H functionalizations of benzoic acid derivatives. (a) Previous reports onmeta-C–H functionalizations of limited benzoic acid derivatives. (b) Our design of template formeta-C–H functionalizations of electron-poor benzoic acid derivatives and the highlights of our work. (c) Representative drugs of benzoic acid derivatives withmeta-substituents. Figure 1: Transition-metal-catalysed meta -C–H functionalizations of benzoic acid derivatives. ( a ) Previous reports on meta -C–H functionalizations of limited benzoic acid derivatives. ( b ) Our design of template for meta -C–H functionalizations of electron-poor benzoic acid derivatives and the highlights of our work. ( c ) Representative drugs of benzoic acid derivatives with meta -substituents. Full size image Controlling the site-selectivity of C–H activation reactions is an outstanding challenge in the development syntheticially useful C–H functinalization methodology [26] , [27] . So far only a limited number of approaches are available for addressing meta -C–H functionalizations of arenes [28] , [29] , [30] , [31] , [32] , [33] , [34] , [35] , [36] , [37] , [38] , [39] , [40] , [41] , [42] , [43] , [44] , [45] , [46] , [47] , [48] , [49] , [50] , [51] , [52] , [53] , [54] , [55] , [56] , [57] , [58] , [59] , [60] , [61] , [62] , [63] . These approaches include inherent substrate control via steric and/or electronic factors [28] , [29] , [30] , [31] , [32] , [33] , [34] , [35] , chelating group-assisted Cu(II)-catalysed arylation [36] , [37] , ruthenium(II) complex facilitated meta -C–H functionalizations [38] , [39] , [40] , [41] , [42] , [43] , the use of transient norbornene mediator [44] , [45] and formal meta -C–H functionalizations utilizing traceless directing groups [46] , [47] , [48] , [49] , [50] , [51] . Another unique method is the use of nitrile-based templates for meta -C–H functionalizations of electron-rich arenes, such as hydrocinnamic acids and phenylacetic acids, which was pioneered by the group of Yu [54] , [55] , [56] , [57] , [58] , [59] , [60] , [61] , [62] , [63] . However, chelation-assisted meta -C–H activation of electron-poor arenes such as benzoic acid derivatives remains a formidable challenge, possibly due to the low reactivity of the electron-poor arenes towards palladation in this type of C–H activation. Herein, we disclose our discovery of a recyclable nitrile-based sulfonamide template that promotes the olefination and acetoxylation of meta -C–H bonds of a broad range of benzoic acid derivatives ( Fig. 1b ). Notably, a protocol is developed that enables the use of environmentally benign molecular oxygen as the terminal oxidant for chelation-assisted meta -C–H olefination, which previously required the use of costly silver salt oxidants. Development of meta -C–H olefination reaction conditions As benzoic acids are both electronically and structurally distinct from other electron-rich arenes that undergo template-assisted meta -C–H functinalizations, the elaboration of a compatible template-directing group is required to accommodate their unique properties. After investigating several newly designed templates (see Supplementary Table 1 for details ), we found amide 1a bearing a highly electron-withdrawing nosyl group was the most promising substrate. After 1a was subjected to the similar reaction conditions that were developed by us for meta -C–H olefination [64] , [65] , [66] , [67] of phenylethylamines [63] , much to our delight, excellent yields of desired products were obtained with tiny traces of other olefinated isomers ( Table 1 , entry 1). To avoid using the costly silver acetate as the oxidant, we continued to optimize the reaction conditions to search for a less costly oxidant. After screening a few inorganic as well as organic oxidants (entries 2–5), we were very surprised to find Cu(OAc) 2 , which might compete with Pd(OAc) 2 in coordination with the weakly coordinating nitrile group, could be used as an effective oxidant (entry 2). The yield was increased to 72% when the reaction was run under oxygen atmosphere (entry 6) [10] , [68] , [69] . Notably, better results were obtained by increasing the loading of Ac-Gly-OH ligand (entries 7–8), leading to almost full conversion of the substrate with 60 mol% of the ligand (entry 8). By further tuning the loading of Cu(OAc) 2 , the reaction time and temperature (entries 9–13), the best result was achieved in 48 h at 90 °C using oxygen as the terminal oxidant with catalytic amount of Cu(OAc) 2 (entry 13). It was found that the reaction was almost shut down without adding Cu(OAc) 2 as co-oxidant (entry 12). The use of oxygen is notable as all the previous chelation-assisted meta -C–H olefination reactions required the use of silver salt as the oxidant [54] , [55] , [56] , [57] , [58] , [59] , [60] , [61] , [62] , [63] . Finally, the reaction conditions were carefully tuned to improve the mono versus di-olefination selectivity (see also Supplementary Table 1 for details ), although the two products could be easily separated. Pleasingly, the use of Formyl-Gly-OH ligand with an inorganic base would result in good mono versus di-olefination selectivities (entries 14–15) [59] , albeit in lower overall yield. Interestingly, this selectivity was switched when no inorganic base was added (entry 16). Table 1 Optimization of reaction conditions. Full size table Substrate scope of meta -C–H olefination With the optimized conditions in hand, we carried out olefinations on a variety of benzoic acid derivatives, which were easily prepared in one step from benzoic acids using routine conditions (see Supplementary Methods for details ). It was found that both electron-donating and electron-withdrawing ortho -substituents were well tolerated ( Fig. 2a , 3b – 3e ), and a good yield of mono-olefinated product was obtained with substrate 1b . Di-olefination occurred predominantly with less hindered amides 1c – 1e . Notably, our method provided a direct access to an aspirin derivative ( 3e ). The reaction also proceeded smoothly with meta -substituted substrates ( 3f – 3h ). Para -substituted benzamides with electron-donating methoxy ( 3i ) and methyl ( 3j ) groups as well as electron-withdrawing fluoro ( 3k ), chloro ( 3l ) and bromo ( 3m ) groups were all suitable substrates, affording mono-olefinated products selectively. Interesting, the bromo group ( 3m ) was tolerated in our protocol, which is synthetically useful for further elaborations of the product. It should be noted di-olefination products with high overall yields could also be produced when KH 2 PO 4 was used as the base for substrates 1j – 1l (see Supplementary Methods for details ). Importantly, the method was compatible with a range of substrates carrying two substituents ( 3n – 3w ), generally producing high yields of desired products. It is surprising that tri-substituted substrates were also able to afford desired products in moderate to high yields ( 3x – 3z ). Such highly substituted patterns were not observed in all previous transition-metal catalysed meta -C–H functionalizations. Desired products were also generated with other electron-deficient olefin-coupling partners ( 3fa – 3fe ), although production of 3fc and 3fd required silver acetate as the oxidant since the standard conditions only afforded low yields of these two products. The meta -selectivity was generally excellent, although traces of isomers were observed for some substrates. However, it was hard to assign the peaks of isomers that were only traces from the crude 1 H NMR and thus we did not attempt to calculate the exact ratios of isomers. Finally, the template-directing group could be removed and recycled readily with LiOH or K 2 CO 3 in high yields as shown in Fig. 2b . Moreover, the auxiliary 5 could be synthesized in multi-gram scale from inexpensive chemicals (see Supplementary Methods for details ). 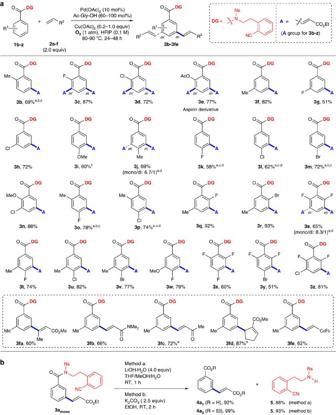Figure 2: Substrate scope and removal and recycle of the template. (a) Substrate scope ofmeta-C–H olefination. Reaction conditions:1(0.1–0.2 mmol),2(2.0 equiv), Pd(OAc)2(10 mol%), Ac-Gly-OH (60–100 mol%), Cu(OAc)2(0.2–1.0 equiv), O2(1 atm), HFIP (1–2 ml), 80–90 °C, 24–48 h, see theSupplementary Methodsfor details. Isolated yields are reported.aFormyl-Gly-OH (60 mol%) was used instead of Ac-Gly-OH.bKH2PO4(0.5 equiv) was added.cA trace of (m,m')-diolefinated product was observed.dK2HPO4(0.5 equiv) was added.eAgOAc (3.0 equiv) was used instead of O2/Cu(OAc)2. (b) Two mild methods available for regenerating auxiliary5. Figure 2: Substrate scope and removal and recycle of the template. ( a ) Substrate scope of meta -C–H olefination. Reaction conditions: 1 (0.1–0.2 mmol), 2 (2.0 equiv), Pd(OAc) 2 (10 mol%), Ac-Gly-OH (60–100 mol%), Cu(OAc) 2 (0.2–1.0 equiv), O 2 (1 atm), HFIP (1–2 ml), 80–90 °C, 24–48 h, see the Supplementary Methods for details. Isolated yields are reported. a Formyl-Gly-OH (60 mol%) was used instead of Ac-Gly-OH. b KH 2 PO 4 (0.5 equiv) was added. c A trace of ( m,m' )-diolefinated product was observed. d K 2 HPO 4 (0.5 equiv) was added. e AgOAc (3.0 equiv) was used instead of O 2 /Cu(OAc) 2 . ( b ) Two mild methods available for regenerating auxiliary 5 . Full size image Meta -C–H acetoxylation The versatility of our sulfonamide template with different catalytic cycles was investigated briefly with meta -acetoxylation of benzoic acid derivatives using the previously established oxidation conditions ( Fig. 3a ) [70] . Although the acetoxylation was generally less efficient than olefination, several substrates with different substitution patterns underwent meta -acetoxylation successfully to give desired products in moderate to good yields ( 6a–6za ). Moreover, 60% combined yield of products was obtained when the reaction was performed in 1.3 mmol scale ( 6a ). 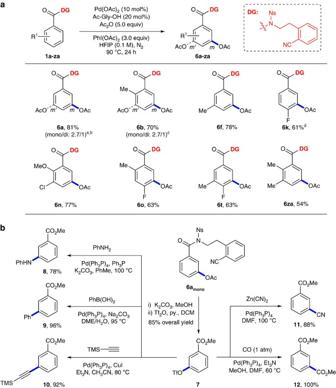Figure 3:Meta-C–H acetoxylation and synthetic elaboration. (a)Meta-C–H acetoxylation. Reaction conditions:1(0.1 mmol), Pd(OAc)2(10 mol%), Ac-Gly-OH (20 mol%), Ac2O (5.0 equiv), PhI(OAc)2(3.0 equiv), HFIP (1 ml), N2, 90 °C, 24 h. Isolated yields are reported; see theSupplementary Methodsfor details.aA trace of regioisomer was observed.bThe yield was 60% (mono/di: 4.8:1) in 1.3 mmol scale.c6 h.dA trace of (m,m')-di-acetoxylated product was observed. (b) Application potential ofmeta-acetoxylation demonstrated with further elaborations. Figure 3: Meta -C–H acetoxylation and synthetic elaboration. ( a ) Meta -C–H acetoxylation. Reaction conditions: 1 (0.1 mmol), Pd(OAc) 2 (10 mol%), Ac-Gly-OH (20 mol%), Ac 2 O (5.0 equiv), PhI(OAc) 2 (3.0 equiv), HFIP (1 ml), N 2 , 90 °C, 24 h. Isolated yields are reported; see the Supplementary Methods for details. a A trace of regioisomer was observed. b The yield was 60% (mono/di: 4.8:1) in 1.3 mmol scale. c 6 h. d A trace of ( m,m' )-di-acetoxylated product was observed. ( b ) Application potential of meta -acetoxylation demonstrated with further elaborations. Full size image Synthetic elaboration To demonstrate the utility of our meta -C–H functionalizations, we attempted further elaboration of the acetoxylated product ( Fig. 3b ). Thus, triflate 7 was prepared in high yield from 6a mono by hydrolysis of the template and the acetoxy group in one step, which was followed by triflation of the resulting hydroxyl group. Triflate 7 was then transformed to a range of synthetically useful substances with well-established coupling reactions, namely, amination ( 8 ), arylation ( 9 ), alkynylation ( 10 ), cyanation ( 11 ) and carbonylation ( 12 ), greatly expanding the application potential of our method. Proposed catalytic cycle On the basis of the above results, a plausible catalytic cycle is proposed for meta -C–H olefination ( Fig. 4 ). The complex A is generated by coordination of substrate 1 to a Pd(II) species followed by template-directed insertion of Pd(II) into the meta -C–H bond of 1 . Following coordination of A with olefin 2 , the resulting complex B undergoes 1,2-migratory insertion to give intermediate C . Product 3 is then afforded by β -hydride elimination of C . Reductive elimination of hydride D produces Pd(0), which is reoxidized to Pd(II) by two equivalents of Cu(II). The resulting Cu(I) is then oxidized by molecular oxygen to re-enter the catalytic cycle. 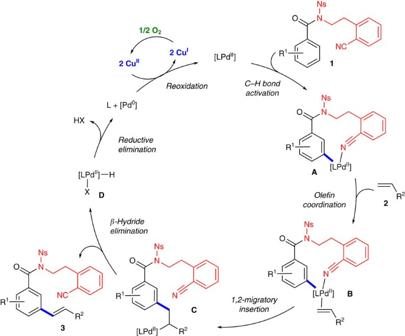Figure 4: Proposed catalytic cycle ofmeta-C–H olefination. The plausible mechanism involves regeneration of a Pd(II) catalyst with only catalytic amount of Cu(II) species. Figure 4: Proposed catalytic cycle of meta -C–H olefination. The plausible mechanism involves regeneration of a Pd(II) catalyst with only catalytic amount of Cu(II) species. Full size image In summary, a general protocol for meta -C–H bond olefination of a broad range of benzoic acid derivatives assisted by a nitrile-based sulfonamide template has been developed. Desired meta -functionalized products were obtained regardless of the substitution patterns and steric biases of the substrates. Notably, the challenging tri-substituted substrates were tolerated, which was not observed in previous transition-metal catalysed meta -C–H functionalizations [15] , [16] , [17] , [18] , [19] , [20] , [21] , [22] , [23] , [24] , [25] , [26] , [27] , [28] , [29] , [30] , [31] , [32] , [33] , [34] , [35] , [36] , [37] , [38] , [39] , [40] , [41] , [42] , [43] , [44] , [45] , [46] , [47] , [48] , [49] , [50] , [51] , [52] , [53] , [54] , [55] , [56] , [57] , [58] , [59] , [60] , [61] , [62] , [63] . Importantly, the new protocol was compatible with molecular oxygen as the terminal oxidant. Moreover, the sulfonamide template auxiliary could be efficiently removed and recycled under mild conditions. Finally, the versatility of our template was demonstrated with meta -C–H acetoxylation, which enabled the access to five synthetically useful major classes of substitents at the meta -position of benzoic acid derivatives. It is expected that the protocol disclosed herein will soon inspire the development of more synthetically useful meta -C–H transformations for benzoic acid derivatives. General methods For 1 H and 13 C NMR spectra of compounds in this manuscript and details of the synthetic procedures, see Supplementary Figs 1–102 and Supplementary Methods . General procedure for meta -C–H olefination To a 50-ml Schlenk sealed tube (with a Teflon cap) equipped with a magnetic stir bar was charged with amide 1 (0.10 mmol, 1.0 equiv), Pd(OAc) 2 (2.3 mg, 0.010 mmol, 10 mol%), Ac-Gly-OH (20–100 mol%) and Cu(OAc) 2 (0.2–1.0 equiv) sequentially. Hexafluoro-2-propanol (HFIP; 1.0 ml) was added to the mixture along the inside wall of the tube, followed by the corresponding alkene 2 (2.0 equiv). The reaction tube was capped, then evacuated briefly under vacuum and charged with O 2 (1 atm, balloon, × 3). The tube was then submerged into a preheated 80 or 90 °C oil bath. The reaction was stirred for 24–48 h and cooled to room temperature. The crude reaction mixture was diluted with EtOAc (5 ml) and filtered through a short pad of Celite. The sealed tube and Celite pad were washed with an additional 20 ml of EtOAc. The filtrate was concentrated in vacuo , and the resulting residue was purified by flash silica gel chromatography or preparative thin layer chromatography using petroleum ether/EtOAc as the eluent. The site selectivity was assigned by NMR analysis of the product or the hydrolysed product. Full experimental details and characterization of new compounds can be found in the Supplementary Methods . General procedure for meta -C–H acetoxylation To a 50-ml Schlenk sealed tube (with a Teflon cap) equipped with a magnetic stir bar was charged with amide 1 (0.10 mmol, 1.0 equiv), Pd(OAc) 2 (2.3 mg, 0.010 mmol, 10 mol%), Ac-Gly-OH (2.4 mg, 0.020 mmol, 20 mol%) and PhI(OAc) 2 (96.6 mg, 0.30 mmol, 3 equiv). HFIP (1.0 ml) was added to the mixture along the inside wall of the tube, followed by Ac 2 O (47 μl, 5 equiv). The reaction tube was capped, then evacuated briefly under vacuum and charged with N 2 (1 atm, balloon, × 3). The tube was then submerged into a preheated 90 °C oil bath. The reaction was stirred for 24 h and cooled to room temperature. The crude reaction mixture was diluted with EtOAc (5 ml) and filtered through a short pad of Celite. The sealed tube and Celite pad were washed with an additional 20 ml of EtOAc. The filtrate was concentrated in vacuo , and the resulting residue was purified by flash silica gel chromatography using petroleum ether/EtOAc as the eluent. Full experimental details and characterization of new compounds can be found in the Supplementary Methods . How to cite this article: Li, S. et al . Pd(II)-catalysed meta -C–H functionalizations of benzoic acid derivatives. Nat. Commun . 7:10443 doi: 10.1038/ncomms10443 (2016).